Uncovering many-body correlations in nanoscale nuclear spin baths by central spin decoherence Central spin decoherence caused by nuclear spin baths is often a critical issue in various quantum computing schemes, and it has also been used for sensing single-nuclear spins. Recent theoretical studies suggest that central spin decoherence can act as a probe of many-body physics in spin baths; however, identification and detection of many-body correlations of nuclear spins in nanoscale systems are highly challenging. Here, taking a phosphorus donor electron spin in a 29 Si nuclear spin bath as our model system, we discover both theoretically and experimentally that many-body correlations in nanoscale nuclear spin baths produce identifiable signatures in decoherence of the central spin under multiple-pulse dynamical decoupling control. We demonstrate that under control by an odd or even number of pulses, the central spin decoherence is principally caused by second- or fourth-order nuclear spin correlations, respectively. This study marks an important step toward studying many-body physics using spin qubits. Decoherence of a central spin in a solid-state environment is not only an ideal model problem for understanding the foundation of quantum physics [1] , [2] , [3] , but also a critical issue in a number of quantum technologies including spin-based quantum information processing [4] , [5] and ultrasensitive magnetometry [6] , [7] , [8] , [9] , [10] . For example, decoherence from the environmental spin bath is often a limiting factor when using systems such as phosphorous donors in silicon [11] , [12] , [13] , [14] , [15] , [16] , semiconductor quantum dots [17] , [18] and nitrogen vacancy centres in diamond [19] , [20] , as quantum bits or sensors. Studying central spin decoherence caused by environmental fluctuations or elementary excitations may yield key insights into the nature of many-body interactions in the environment. Furthermore, dynamical control over the central spin can affect the dynamics of the environment in a detectable manner [8] , [18] , even to the extent of coherently controlling [21] , [22] or dynamically polarizing nuclear spin baths [23] , [24] . In the light of these ideas, exploiting central spin decoherence for sensing single-nuclear spins or nuclear spin clusters in spin baths has been theoretically proposed [6] , [7] , [8] and experimentally demonstrated [9] , [10] . Recently, this idea has been pushed to new depths: theoretical studies show that the central spin decoherence can be a novel probe to many-body physics, in particular, phase transitions in spin baths [25] , [26] , [27] , [28] . Multiple-spin correlations are one of the essential characteristics in spin baths [11] , [12] , [13] , [14] , [15] , [16] , [17] , [18] , [19] , [20] , but detection of such correlations is a long-standing challenge in many-body physics. Here we address this problem with the first experimental demonstration of detection of many-body correlations via central spin decoherence, laying a foundation for studying many-body physics and phase transitions in spin baths [25] , [26] , [27] , [28] . Previous approaches to studying multiple-particle correlations include the use of nonlinear optical spectroscopy of excitons in semiconductors [29] , [30] , [31] , [32] , nuclear magnetic resonance (NMR) spectroscopy of nuclear spins in molecules [33] , and the generalization of multi-dimensional NMR to optical spectroscopy [34] , [35] . Nevertheless, the detection and characterization of many-body correlations in nanoscale systems [36] , [37] remain highly challenging due to the weak signals in such small systems. In this article, taking a phosphorus donor electron spin in a natural-abundance 29 Si nuclear spin bath as our model system, we show both theoretically and experimentally that many-body correlations in nanoscale nuclear spin baths produce identifiable signatures in the decoherence of the central spin under multiple-pulse dynamical decoupling (DD) control. The DD control over the central spin establishes and manipulates correlations among the nuclear spins in the bath. When the number of decoupling π -pulses is odd, central spin decoherence is primarily driven by second-order nuclear spin correlations (pairwise flip-flop processes). In contrast, when the number of π -pulses is even, fourth-order nuclear spin correlations (diagonal interaction renormalized pairwise flip-flop processes) are principally responsible for the central spin decoherence. Our method is particularly suited for the detection of many-body correlations in nanoscale systems. System and model We consider the electron spin ( S =1/2) of a phosphorus donor localized in silicon as the central spin ( Fig. 1a ). This donor electron spin is coupled with a 29 Si nuclear spin bath ( I =1/2 and natural abundance of 4.7% throughout the host lattice) by the contact hyperfine interactions and dipolar interactions [14] . 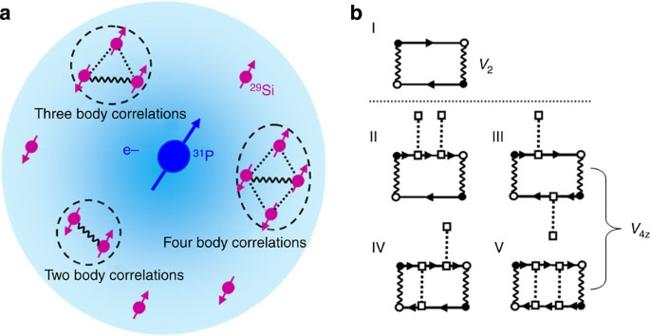Figure 1: Many-body correlations in the29Si nuclear spin bath probed by a phosphorus donor electron spin. (a) Due to the extended donor wavefunction, the P-donor electron spin (blue arrow) interacts with a bath of29Si nuclear spins (magenta arrows) possessing various many-body correlations. (b) Topologically inequivalent connected diagrams (LCE diagrams) corresponding to different many-body correlations in the nuclear spin bath: (I)V2—second-order pairwise flip-flop diagram, (II–V)V4z—fourth-order diagonal interaction renormalized pairwise flip-flop diagrams. Here the nuclear spin operatorsare represented in turn by filled circles, empty circles or empty squares. The off-diagonal (diagonal) interaction terms are represented by wavy (dashed) lines. The solid arrows represent nuclear spin correlation functions betweenand(or) with the arrows indicating the direction of time propagation. In a strong external magnetic field (>100 mT), the Zeeman energies of the donor spin and nuclear spins are conserved, so the total spin Hamiltonian can be written in the secular form [12] , [13] Figure 1: Many-body correlations in the 29 Si nuclear spin bath probed by a phosphorus donor electron spin. ( a ) Due to the extended donor wavefunction, the P-donor electron spin (blue arrow) interacts with a bath of 29 Si nuclear spins (magenta arrows) possessing various many-body correlations. ( b ) Topologically inequivalent connected diagrams (LCE diagrams) corresponding to different many-body correlations in the nuclear spin bath: (I) V 2 —second-order pairwise flip-flop diagram, (II–V) V 4 z —fourth-order diagonal interaction renormalized pairwise flip-flop diagrams. Here the nuclear spin operators are represented in turn by filled circles, empty circles or empty squares. The off-diagonal (diagonal) interaction terms are represented by wavy (dashed) lines. The solid arrows represent nuclear spin correlation functions between and (or ) with the arrows indicating the direction of time propagation. Full size image where ω e/n = γ e/n B is the Larmor frequency of the donor electron spin /bath nuclear spins, γ e/n is the gyromagnetic ratio of the donor electron spin /bath nuclear spins, and B is the external magnetic field applied along the z axis. The coupling coefficient between the donor spin and the i th nuclear spin is A i = γ e γ n {8 π /3| ψ ( R i )| 2 +∫ d 3 r | ψ ( r )| 2 [3( r z – R i z ) 2 –| r – R i | 2 ]/| r – R i | 5 }, where the first term is the Fermi contact interaction given by the donor electron density | ψ ( R i )| 2 at the position of the i th nuclear spin [14] and the second term is the dipolar interaction. The donor electron density decays exponentially with r , while the dipolor interaction decays with distance by r −3 , such that the dipolar interaction starts contributing only for | R i |> r 0 =2 nm. It can therefore be approximated as γ e γ n θ (| R i |– r 0 )(3cos 2 θ i –1)/| R i | 3 , where θ ( r ) is the Heaviside step function and θ i is the angle between the nuclear spin position vector R i and the magnetic field vector B . The dipolar interaction between the nuclear spins is D ij = γ n 2 (3cos 2 θ ij –1)/4| R ij | 3 , where θ ij is the angle between R ij = R i – R j and B . We assume that the donor electron spin is initially prepared in the coherent state by a π /2 rotation (with +/− being spin-up/down along the magnetic field direction). In the subsequent evolution, the central spin suffers decoherence as a result of its coupling to the nuclear spin bath. However, by applying DD control [38] , [39] to the central spin (consisting of a sequence of π -flips at times { t 1 , t 2 ⋯ t n }), we can reduce its sensitivity to the bath in general while selectively enhancing the effect of certain multiple-spin dynamics [8] . With DD, the restored central spin coherence following a total evolution time T is with P J being the probability of the nuclear state | J › and where H 0 =(1/2)∑ i A i I i z and V =∑ i < j D ij ( I i + I j − + I i − I j + –4 I i z I j z ). Here, the nuclear Zeeman term ω n ∑ i I i z is dropped since it has no contribution to the spin decoherence. The nuclear spin bath is assumed to be in an infinite-temperature (fully mixed) state ( P J =1/2 M ) with density matrix , where | J › is an eigenstate of ∑ i I i z and M being the number of nuclear spins in the bath. We consider two families of DD sequences: Carr–Purcell–Meiboom–Gill (CPMG) [40] , [41] , [42] and Uhrig DD (UDD) [43] , [44] ( Fig. 2a ). An n -pulse CPMG sequence periodically flips the central spin at time t c =(2 c –1) T /2 n , while n -pulse UDD flips the central spin at time t c = T sin 2 [ cπ /(2 n +2)], where T is the total evolution time and c =1, 2, ⋯ , n . It should be noted that CPMG and UDD are equivalent for n ≤2, and for n =1 simply correspond to the Hahn echo. 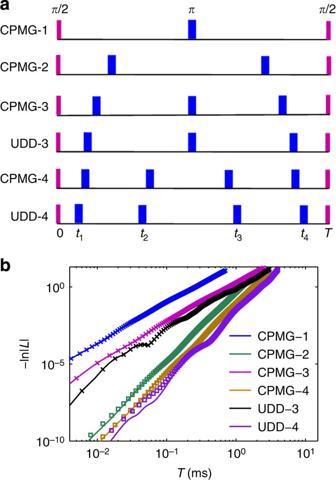Figure 2: Effects of different orders of many-body correlations on central spin decoherence under dynamical decoupling. (a) Schematics of various CPMG and UDD pulse sequences. (b) Comparisons of the P-donor electron spin decoherence in a natural abundance29Si nuclear spin bath calculated by the numerically exact CCE method (lines) and those by the LCE approximation (symbols) to determine the many-body correlations that contribute significantly to the spin decoherence under various CPMG and UDD controls. Here, LCE-V2(crosses) represents the leading-order pairwise flip-flop processes in the nuclear spin bath which dominate for sequences with an odd number ofπpulses, while LCE-V4z(squares) represents the diagonal interaction renormalized pairwise flip-flop processes which dominate for the even-numbered sequences where LCE-V2is zero (seeFig. 1b). The magnetic field was set asB=0.3 T applied along the [110] lattice direction. Figure 2: Effects of different orders of many-body correlations on central spin decoherence under dynamical decoupling. ( a ) Schematics of various CPMG and UDD pulse sequences. ( b ) Comparisons of the P-donor electron spin decoherence in a natural abundance 29 Si nuclear spin bath calculated by the numerically exact CCE method (lines) and those by the LCE approximation (symbols) to determine the many-body correlations that contribute significantly to the spin decoherence under various CPMG and UDD controls. Here, LCE- V 2 (crosses) represents the leading-order pairwise flip-flop processes in the nuclear spin bath which dominate for sequences with an odd number of π pulses, while LCE- V 4 z (squares) represents the diagonal interaction renormalized pairwise flip-flop processes which dominate for the even-numbered sequences where LCE- V 2 is zero (see Fig. 1b ). The magnetic field was set as B =0.3 T applied along the [110] lattice direction. Full size image Many-body correlation effects on central spin decoherence According to the linked-cluster expansion (LCE) theorem in many-body physics [45] , the quantum evolution of a nuclear spin bath from an initial state | J › can be factorized into contributions of different orders of irreducible many-body correlations, namely, with the l th order many-body correlation where is the time-ordering operator along the contour C (0→ T →0), and V ( t )=exp( iH 0 t ) V exp(− iH 0 t ) is the intra-bath coupling in the interaction picture. Note that the hyperfine interaction H 0 enters into the time evolution of the bath correlations. We show some examples of the expansion terms diagrammatically in Fig. 1b (see Methods for calculation of the diagrams). Here we assume the nuclear spin bath starts from a pure product state | J ›. The thermal ensemble results can be obtained by sampling over different initial states and then taking a statistical average. For each LCE term, the real part contributes to the spin decoherence while the imaginary part just produces a coherent phase shift (corresponding to self-energy renormalization of the probe spin). Under CPMG- n or UDD- n control, the first-order LCE term ( l =1) vanishes due to the contour integral. The second-order LCE term ( l =2) corresponds to the leading-order pairwise flip-flop processes in the nuclear spin bath, in which the bath dynamics is approximated as a product of evolutions of nuclear spin pairs [15] , [17] , [18] . Previous studies identified this term as the main cause of spin decoherence for the free-induction decay and Hahn echo in the strong magnetic field regime [15] , [17] , [18] . The pairwise flip-flop processes of nuclear spins i , j can be mapped to the precession of a pseudospin σ ij about a pseudofield =( D ij , 0, ± ω ij /2) conditioned on the central spin state |±› (ref. 17 ), where ω ij =( A i − A j )/2 is the energy cost of the flip-flop process (see ‘Pseudospin model’ in Methods for details). If the central spin is under CPMG- n control, we have when n is odd, but when n is even (see the schematics in Fig. 3a ), where t = T /2 n . For UDD- n control, the real part of the second-order LCE term also vanishes when n is even and is non-zero when n is odd (see ‘Derivation of LCE terms’ in Methods for details). 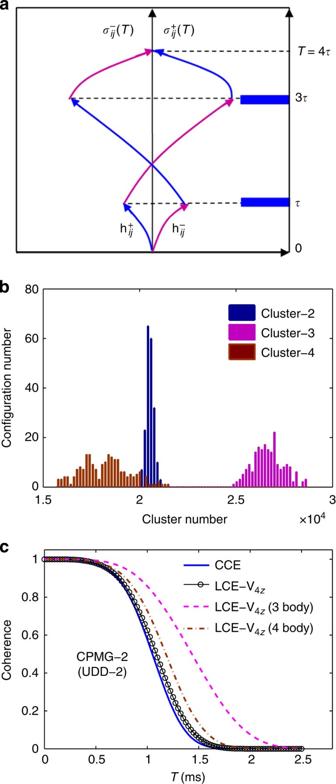Figure 3: Contributions of three-body and four-body correlations to the central spin decoherence under CPMG-2 control. (a) Schematics of bifurcated pseudospin evolutions conditioned on the central spin state under CPMG-2 (or UDD-2) control. The conjugate pseudospins(corresponding to the central spin in the state |±›) describe the dynamics of two-spin correlations. The more the trajectories are separated, the greater the central spin decoherence. The conjugate pseudospins exchange their pseudofieldsat timet=τ, 3τwhen the central spin is flipped by aπ-pulse. Without the diagonal interaction renormalization, the conjugate trajectories are symmetric and coincide at timeTin the leading order of the evolution time, leading to cancellation of decoherence. (b) Histogram of the number of nuclear spin clusters (with inter-nuclei distances <1 nm) in 200 different bath configurations. (c) Decomposition of the LCE-V4zterm into three-body and four-body correlations (seeFig. 1a) for CPMG-2 (or UDD-2) control of the central spin. The magnetic field wasB=0.3 T applied along the [110] lattice direction. Figure 3: Contributions of three-body and four-body correlations to the central spin decoherence under CPMG-2 control. ( a ) Schematics of bifurcated pseudospin evolutions conditioned on the central spin state under CPMG-2 (or UDD-2) control. The conjugate pseudospins (corresponding to the central spin in the state |±›) describe the dynamics of two-spin correlations. The more the trajectories are separated, the greater the central spin decoherence. The conjugate pseudospins exchange their pseudofields at time t = τ , 3 τ when the central spin is flipped by a π -pulse. Without the diagonal interaction renormalization, the conjugate trajectories are symmetric and coincide at time T in the leading order of the evolution time, leading to cancellation of decoherence. ( b ) Histogram of the number of nuclear spin clusters (with inter-nuclei distances <1 nm) in 200 different bath configurations. ( c ) Decomposition of the LCE- V 4 z term into three-body and four-body correlations (see Fig. 1a ) for CPMG-2 (or UDD-2) control of the central spin. The magnetic field was B =0.3 T applied along the [110] lattice direction. Full size image For higher order LCE terms, there are three groups of diagrams: ring diagrams, diagonal-interaction renormalized diagrams and locked diagrams [45] . Generally, the leading terms of the l th order diagrams are proportional to ( D ij / ω ij ) l . Due to the random distribution of nuclear spins, the contributions from different nuclear spin clusters add destructively when l is odd but add constructively when l is even. Hence, the odd-order LCE terms contribute negligibly to the spin decoherence. The central spin decoherence problem can be exactly solved by the cluster-correlation expansion (CCE) method [46] . To identify the contributions of different many-body correlations to the central spin decoherence, we compare the approximate results obtained by the LCE to the exact numerical results obtained by the CCE ( Fig. 2b ). We see that the second-order pairwise flip-flop LCE term ( V 2 ) almost fully reproduces the CCE results for DD controls of odd pulse number, while the contribution of the fourth-order diagonal-interaction renormalized LCE term ( V 4 z ) coincides with the CCE results for DD controls of even pulse number. This indicates that we can selectively detect either the second-order or fourth-order many-body correlations by choosing an appropriate number of DD control pulses. Similar pulse-number parity effects were theoretically noticed before [42] , however, without analysing the underlying microscopic processes. The different correlations actually present different central spin decoherence features. In particular, the V 2 correlation causes decoherence with a faster initial decay but a longer decay tail ( ); while the decoherence induced by the V 4 z correlation is better preserved in the short time regime but decays faster in the long time regime ( ). It should be pointed out that the LCE- V 4 z term contains two-body, three-body and four-body nuclear spin correlations ( Fig. 1b ). The two-body V 4 z correlations have no contribution to decoherence, because the pairwise flip-flop of two nuclear spins is independent of the diagonal interaction between them. The nuclear spin clusters contributing the most to central spin decoherence are those four-spin or three-spin clusters with small inter-nuclei distances (<1 nm), so that the energy cost of the pairwise flip-flop processes of two nuclear spins is significantly changed by the other nuclear spins in the cluster (see ‘Pseudospin model’ in Methods for details). The typical strength of the interaction between nuclear spins in such clusters is ~100 Hz, which is in the same order of the NMR linewidth of 29 Si in natural silicon samples [23] . In the calculations, we consider a bath volume with radius 8 nm from the central spin, corresponding to 5,000 nuclear spins. Statistical studies ( Fig. 3b ) show that there are about 1.8 × 10 4 such four-spin clusters and 2.6 × 10 4 three-spin clusters in the bath. In Fig. 3c , we compare the contributions of different many-body correlations and find that the four-body correlations are the main contribution to the central spin decoherence under DD control of even number of pulses. The three-body correlations are non-zero but relatively small. Experimental results We have observed the pulse-number parity effect in DD experiments on P-donors in natural Si ( Fig. 4 ). The measured decoherence decays fit well in stretched exponential functions (see Supplementary Fig. 1 ). Here the first term represents the instantaneous diffusion caused by dipolar coupling to other P-donor electron spins in the sample ([P]=3 × 10 14 per cm 3 ), and the second term represents the central spin decoherence (spectral diffusion) caused by the 29 Si nuclear spin bath. 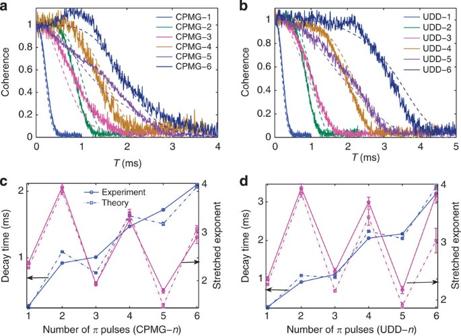Figure 4: Comparison between theoretical and experimental results ofnatSi:P electron spin decoherence under dynamical decoupling. (a,b) Measured (solid lines) and calculated (dashed lines) coherence of the P-donor electron spin in the natural29Si nuclear spin bath under (a) CPMG or (b) UDD control. We attribute the deviation seen at ~1 ms for CPMG-6 to an overlap with uncorrected stimulated/unwanted echoes. (c,d) Comparisons of the experimental (solid lines) and theoretical (dashed line) decay timesτSD(blue) and stretched exponentsλ(magenta) of the central spin decoherence under (c) CPMG or (d) UDD control. The error bars correspond to the systematic errors of the stretched exponential fitting of the plots ina,b. The magnetic field wasB=0.3 T applied along the [110] lattice direction. Figure 4: Comparison between theoretical and experimental results of nat Si:P electron spin decoherence under dynamical decoupling. ( a , b ) Measured (solid lines) and calculated (dashed lines) coherence of the P-donor electron spin in the natural 29 Si nuclear spin bath under ( a ) CPMG or ( b ) UDD control. We attribute the deviation seen at ~1 ms for CPMG-6 to an overlap with uncorrected stimulated/unwanted echoes. ( c , d ) Comparisons of the experimental (solid lines) and theoretical (dashed line) decay times τ SD (blue) and stretched exponents λ (magenta) of the central spin decoherence under ( c ) CPMG or ( d ) UDD control. The error bars correspond to the systematic errors of the stretched exponential fitting of the plots in a , b . The magnetic field was B =0.3 T applied along the [110] lattice direction. Full size image In Fig. 4a,b , we show the measured decays, corrected to exclude the instantaneous diffusion (with τ ID =10 ms determined by the initial exponential decay of the raw experimental data in Supplementary Fig. 1 ). The measured and calculated results agree well for both CPMG- n and UDD- n controls, without any adjustable parameters in the calculations. In Fig. 4c,d , we compare the central spin coherence decay time τ SD and exponent stretching factor λ of the measured and numerical data as functions of the pulse number n . The quantitative and qualitative agreement is remarkable, the only exception being that the measured decay time τ SD oscillates with n somewhat less strongly than expected. As predicted, the stretching factor λ oscillates between about 2 and 4 as n increases, meaning that either the second-order correlations or fourth-order correlations contribute dominantly to central spin decoherence. The slight decrease of the stretched exponent λ with n can be ascribed to the emergence of the ‘Markovian’ decoherence when the coherence time is prolonged to exceed the pairwise flip-flop time and the higher order many-body correlations become more important [46] . The different signatures of the many-body correlations under DD control of the central spin, in particular the pulse-number parity effect in the number of DD control pulses, provide a useful approach to studying many-body physics in the nuclear spin bath. Note that the parity effect is not affected by the type of DD sequences adopted in this paper—it exists in both CPMG and UDD controls. It is remarkable that the many-body correlations between nuclear spins have sizable effects even at temperatures (a few Kelvin in our experiments) much higher than the coupling strengths between the nuclear spins (a few nano-Kelvin). The pulse-number parity effect should be observable in a broad range of central spin systems as long as the following conditions are satisfied: (i) pure dephasing condition—the external magnetic field should be large so that the energy non-conserving processes (such as single-nuclear spin rotations) are highly suppressed (that is, the total Hamiltonian can be written in the secular form); (ii) slow/non-Markovian bath condition—the decoherence time should be much shorter than the nuclear spin cluster correlation times (so that the LCE terms converge rapidly with increasing orders and the central spin decoherence is mainly induced by the lowest-order non-zero LCE terms). Extending the study of nuclear spin correlation effects to other types of shallow donors in semiconductors (such as bismuth donors in silicon [47] , [48] ) would be quite straightforward. It is also possible to observe similar effects for electron spins in semiconductor quantum dots (such as GaAs and InAs quantum dots [17] , [18] , [42] ) under the conditions that a strong magnetic field (>100 mT) is applied and DD control is available. On the other hand, deep centres like nitrogen vacancy centres in diamond are not likely to produce the pulse-parity effect, since in such systems, the electron spins interact with only a small number of nuclear spins (~100) through the (rapidly decaying) dipolar interaction and the decoherence time becomes comparable with the nuclear spin cluster correlation time. This makes the higher order LCE terms (compared with V 2 and V 4 z ) contribute significantly to decoherence for both odd and even pulse numbers. The detection of many-body correlations may find applications in identifying the structures of molecules and defect complexes in solids. For example, the pulse-number parity effect can be adopted to tell whether the molecules/defects that form the nuclear spin bath have two-body or higher order interactions among the nuclei. The delocalized nature of the electron spin in many molecules [49] makes it interact with a large number of nuclear spins and therefore lends itself to such an approach. It should be noted that the current scheme can only detect up to the fourth order (four-body) correlations. Generalization to detection of higher order correlations is in principle possible by using more complicated dynamical control (in timing, composition, and so on) and/or different types of probes (for example, higher spins). Exploration along this line will provide interesting topics for future studies. Interaction picture The propagators of the nuclear spin bath can be written as [45] where is the time-ordering operator and with and ω i = A i /2. By the relations above, the operator can be rewritten in the interaction picture as the product of several evolution operators. For example, for the CPMG-1 (UDD-1) and CPMG-2 (UDD-2) controls with t = T /(2 n ). Generalized Wick’s theorem for spin 1/2 Wick’s theorem for bosons or fermions cannot be directly used for the nuclear spins, because the commutation brackets of spin operators do not yield c-numbers. Previous studies generalized Wick’s theorem to spin 1/2 operators [45] , [50] . First, we define the contraction of two spin operators as where is the normal ordered operator depending on the state of the nuclear spin such that . For example, If the i th nuclear spin is in the spin-down state ( ), we have the following contraction relations [50] where θ ( t ) is the Heaviside step function. If , we can get the new contraction relations from equation (11) by the transformation and with the right side of the equations changing the signs. Now we can state the generalized Wick’s theorem for spin 1/2 operators: the time-ordered product of a set of time-dependent spin operators is equal to the sum of all possible fully contracted products which contains only operators [45] , [50] . Derivation of LCE terms Now we can derive the analytical forms of the LCE terms. First we calculate the LCE- V 1 term ( Fig. 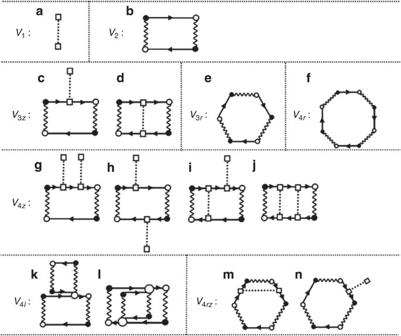Figure 5: LCE diagrams for different many-body correlations in the nuclear spin bath up to the fourth order. (a)V1—first-order diagram, (b)V2—second-order pairwise flip-flop diagram, (c,d)V3z—third-order diagonal interaction renormalized pairwise flip-flop diagrams, (e)V3r—third-order ring diagram, (f)V4r—fourth-order ring diagram, (g–j)V4z—fourth-order diagonal interaction renormalized pairwise flip-flop diagrams, (k,l)V4l—fourth-order locked diagrams.(m,n)V4rz—fourth-order diagonal interaction renormalized ring diagrams. 5a ), Figure 5: LCE diagrams for different many-body correlations in the nuclear spin bath up to the fourth order. ( a ) V 1 —first-order diagram, ( b ) V 2 —second-order pairwise flip-flop diagram, ( c , d ) V 3 z —third-order diagonal interaction renormalized pairwise flip-flop diagrams, ( e ) V 3 r —third-order ring diagram, ( f ) V 4 r —fourth-order ring diagram, ( g – j ) V 4 z —fourth-order diagonal interaction renormalized pairwise flip-flop diagrams, ( k , l ) V 4 l —fourth-order locked diagrams. ( m , n ) V 4 rz —fourth-order diagonal interaction renormalized ring diagrams. Full size image where and . We see that this term vanishes due to the contour integral. The LCE- V 2 term ( Fig. 5b ) is For the CPMG- n control, we have when n is odd, and Re‹ V 2 ›=0 when n is even. For the UDD- n control, we also have Re‹ V 2 ›=0 when n is even, but Re‹ V 2 › cannot be written in a simple compact form as in the CPMG case when n is odd ( n >2). The LCE- V 4 z term includes four diagrams ( Fig. 5g–j ). However, the last two diagrams ( Fig. 5i,j ) have no contribution to central spin decoherence, because the pairwise flip-flop processes of nuclear spins ( i , j ) are independent of the diagonal interactions between them ( ) (so the fourth order terms in Fig. 5i,j approximately reduce to the same form as in Fig. 5c,d , respectively, but are higher order small quantities). Therefore the pairwise dynamics ( Fig. 6a ) is well approximated by the diagram in Fig. 5b . For the diagrams in Fig. 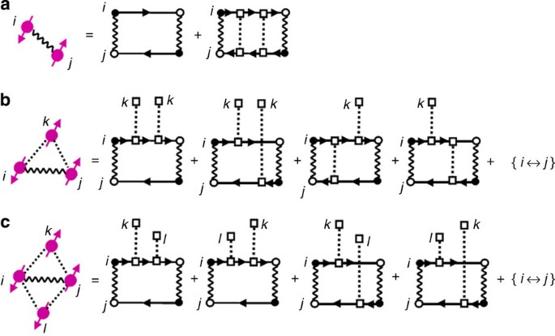Figure 6: Decomposition of many-body correlations into LCE diagrams. We only consider theV2andV4zterms contributing most to central spin decoherence. The fourth-order diagonal-interaction renormalized pair flip-flop processes (V4z) can be two-body, three-body or four-body correlations. The two-body correlations describe the pairwise flip-flop processes of nuclear spinsi,jrenormalized by the diagonal couplings betweeniandj, while the three-body (four-body) correlations describe the pairwise flip-flop processes of nuclear spinsi,jrenormalized by the diagonal couplings ofi,jto nuclear spink(k,l) in the nuclear spin bath. Note that in this figure, the vertices along the same horizontal line are of the same spin. 5g,h , we can get analytical results of the three-body and four-body correlations for the CPMG and UDD control of even pulse number as follows Figure 6: Decomposition of many-body correlations into LCE diagrams. We only consider the V 2 and V 4 z terms contributing most to central spin decoherence. The fourth-order diagonal-interaction renormalized pair flip-flop processes ( V 4 z ) can be two-body, three-body or four-body correlations. The two-body correlations describe the pairwise flip-flop processes of nuclear spins i , j renormalized by the diagonal couplings between i and j , while the three-body (four-body) correlations describe the pairwise flip-flop processes of nuclear spins i , j renormalized by the diagonal couplings of i , j to nuclear spin k ( k , l ) in the nuclear spin bath. Note that in this figure, the vertices along the same horizontal line are of the same spin. Full size image where L ijk and L ijkl denote the central spin decoherence caused by the diagonal interaction renormalized pairwise flip-flop processes ( i ↔ j ) in the three-spin cluster { i , j , k } ( Fig. 6b ) and four-spin clusters { i , j , k , l } ( Fig. 6c ), respectively, and . These analytical expressions imply that to have significant contributions to the central spin decoherence, the nuclear spin clusters should satisfy the following conditions: (i) the inter-nuclei distances in four-spin clusters or three-spin clusters should be rather small (<1 nm); (ii) the renormalization to the energy cost of the pair flip-flop ( i , j ) should be substantial as compared with the bare energy cost, that is, should be large for three-spin clusters { i , j , k } while should be positive and large for four-spin clusters{ i , j , k , l }. Pseudospin model To get an intuitive understanding of the pulse-number parity effect, we use the pseudospin model [17] to describe the dynamics of two nuclear spins. In the strong field regime, the Hamiltonian of the i th and j th nuclear spins conditioned on the central spin state where the basis set is defined as . Note that the two pseudofields corresponding to the two opposite central spin states lie in the xz plane and are symmetric with respect to the x axis. The time evolution operator is Where φ = κt , , , . If the central spin is under CPMG- n or UDD- n control, the time evolution operator can be obtained by the above formula. For CPMG-1 (UDD-1) and CPMG-2 (UDD-2) controls, we have For the donor spin in silicon, we have ω ij ≫ D ij , so n x ≈2 D ij / ω ij is a small quantity. The difference between and causes the central spin decoherence . When n =2 k +1, we have and . However, when n =2 k , due to the symmetry between the two pseudofields corresponding to the two opposite central spin states, the two conjugate trajectories of the pseudospin under the two pseudofields cross into each other (in the leading order of evolution time) at the end of the DD control. Therefore and . Here f n ( T ) is a function of the total evolution time T and the pulse number of DD control n . If we consider all the nuclear spins in the bath, then the central spin decoherence can be expressed as the product of the decoherence contributed by each pair of nuclear spins. Then we have These results are consistent with results obtained by the LCE method. Recall that the LCE- V l terms are proportional to ( D ij / ω ij ) l . Therefore, for CPMG or UDD control of odd pulse numbers, the second-order correlations contribute the most to the central spin decoherence. But for the CPMG or UDD control of even pulse numbers, the second-order correlations are cancelled and the fourth-order correlations corresponding to the ring diagrams V 4 r and locked diagrams V 4 l ( Fig. 5 ) would contribute the most to the central spin decoherence. It should be pointed out that in the discussion above, we have not considered the diagonal interactions between the nuclear spins i , j and other nuclear spins in this pseudospin model. Actually, such diagonal interactions will renormalize the pseudospin Hamiltonian and break the symmetry between the two conjugate pseudofields for the pseudospin. The renormalization effect depends on the magnetic field direction which determines the dipolar interactions between nuclear spins (see Supplementary Fig. 2 ). For B //[111], the nearest neighbour nuclear spins (which contributes most to decoherence) have strong dipolar interactions, which make the pairwise flip-flop processes hard to be renormalized by other spins. But as B //[001] or [110], the nearest neighbour nuclear spins have zero or weak dipolar interactions, rendering the pairwise flip-flop processes easier to be renormalized by other spins. Therefore, when the number of pulses is even, the higher order pairwise flip-flop processes ( V 4 l and V 4 r ) contributes most to the central spin decoherence as B //[111], while the diagonal interaction renormalized pairwise flip-flop processes ( V 4 z ) contribute most to the central spin decoherence as B //[001] or [110]. Numerical simulation method The P-donor electron spin decoherence in a natural abundance 29 Si nuclear spin bath was numerically solved by the well-established CCE method [46] . We included about 5,000 nuclear spins that are located within 8 nm from the P-donor nucleus. Nuclear spins beyond this range have negligible contribution to the central spin decoherence as evidenced by the converged numerical results with increasing bath size. The central spin coherence time depends on the random configuration of 29 Si nuclear spin positions in the lattice. To compare with the experimental results, we ran simulations for 100 random nuclear spin configurations and took the ensemble average of the corresponding time-domain spin coherence. Since the central spin decoherence is almost independent of the initial state of the nuclear spin bath as long as the initial state is roughly unpolarized, we just took a random unpolarized single-sample state | J › (an eigenstate of { I i z }) as the initial state of the nuclear spin bath. Experimental setup Experimental results were measured on a natural silicon Czochralski wafer doped with 3 × 10 14 per cm 3 phosphorus, using an X-band (9.6 GHz) Bruker ELEXSYS 580 spectrometer. All decay times were obtained on the high-field electron spin resonance line ( m I =−1/2) at 3,452 G at 6 K (where the electron spin relaxation processes ( T 1 ≈1 s) did not contribute to decoherence over the timescales considered in this paper). The multiple pulses required for the DD sequences can result in ‘stimulated echoes’, and other unwanted echoes, in the experiment due to pulse infidelities. When such echoes overlap with the desired one (from spin packets which have been flipped by all the π pulses), the experimentally observed decay curves gain unwanted contributions. We therefore cycled the phases of the applied π pulses in such a way as to remove the contribution of all undesired echoes. For UDD, the timings between each pulse are different and most stimulated echoes fall outside the desired one which can then be isolated. For example, the phase cycling sequence for UDD-4 requires simply subtracting the echo from two experiments where the first two pulses are changed from + π to – π and the last two are + π . For CMPG, this is more challenging as the intervals are equal and we did not suppress all possible stimulated echoes for CPMG-5 and CPMG-6. How to cite this article : Ma, W.-L. et al. Uncovering many-body correlations in nanoscale nuclear spin baths by central spin decoherence. Nat. Commun. 5:4822 doi: 10.1038/ncomms5822 (2014).